Imaging the structure of the trimer systems4He3and3He4He2 Helium shows fascinating quantum phenomena unseen in any other element. In its liquid phase, it is the only known superfluid. The smallest aggregates of helium, the dimer (He 2 ) and the trimer (He 3 ) are, in their predicted structure, unique natural quantum objects. While one might intuitively expect the structure of 4 He 3 to be an equilateral triangle, a manifold of predictions on its shape have yielded an ongoing dispute for more than 20 years. These predictions range from 4 He 3 being mainly linear to being mainly an equilateral triangle. Here we show experimental images of the wave functions of 4 He 3 and 3 He 4 He 2 obtained by Coulomb explosion imaging of mass-selected clusters. We propose that 4 He 3 is a structureless random cloud and that 3 He 4 He 2 exists as a quantum halo state. Molecules are often intuitively pictured by ball-and-stick models as having a well-defined structure. The delocalization of the relative position of the atoms dictated by quantum mechanics is usually sufficiently small to justify such structure models. This intuition of being constructed from well-localized subunits can also be applied to more loosely bound aggregates as van der Waals molecules and small rare gas clusters. Ne 3 , for example, is a quite stiff equilateral triangle [1] . Helium is the only element that stands out in this respect (see, for example, a recent review by [2] ). Its clusters still give rise to controversial theoretical debates (see ref. 3 for a review of the literature on this controversy). All other elements in the periodic table have some electrons that are more loosely bound than the two electrons of the helium atom. This makes the helium atom the most unpolarizable element. The van der Waals force between two helium atoms is therefore extremely weak and gives rise to only a shallow potential minimum of −0.947 meV depth at an internuclear distance of 2.96 Å (ref. 4 ). This potential supports one bound state of the dimer 4 He 2 with a binding energy in the order of 10 −7 eV with the exact value still being disputed [4] , [5] , [6] . Substituting one 4 He by the isotope 3 He breaks this weak bond. In addition to its effect on the dimer, the combination of weak van der Waals attraction and small mass of 4 He is also the origin of superfluidity found in bulk and in large clusters of 4 He (ref. 7 ). Helium clusters composed of three atoms are even more intriguing quantum systems. Owing to the very large scattering length (≈10 2 Å) of the helium atom, the isotopically pure 4 He 3 trimer offers a unique atomic system to study the universality of a three-body problem [8] . In addition, it represents the most promising candidate for the Efimov effect in a naturally existing system [9] . By replacing one of the three 4 He atoms by the lighter isotope 3 He, the predicted trimer binding energy reduces by about one order of magnitude with respect to the ≈0.011 meV 4 He 3 binding energy [10] as a result of the increase in zero-point motion [11] , [12] . This feature thus makes the 3 He 4 He 2 trimer the most weakly bound three-body molecule, which also exhibits many similarities to the first excited Efimov state in 4 He 3 . It is a so-called Tango state [13] , [14] where only one out of the three dimer-like subsystems is bound ( 4 He– 4 He). Our knowledge of 4 He 3 today stems almost exclusively from theory. The reason is that traditional experimental approaches to chemical structure determination such as vibrational and rotational spectroscopy cannot be applied to these extremely fragile molecules as the centrifugal force already makes the first excited rotational state unbound. The only experimental technique giving access to some geometrical feature of 4 He 3 is matter wave diffraction [15] , which gives a mean size of Å (ref. 16 ) without providing any further information on the structure. Furthermore, the existence of the isotopic 3 He 4 He 2 trimer has recently been confirmed by means of such matter wave diffraction experiments [17] . Although there is theoretical consensus concerning the floppy nature of both the 4 He 3 and 3 He 4 He 2 molecules, the geometrical shape is a matter of extensive current debates. In the particular case of the 4 He 3 trimer some calculations suggest an equilateral triangular structure [18] , [19] , [20] , while others indicate a significant contribution of linear configurations [21] , [22] . It has also been recently suggested that this controversy is often mislead by drawing false conclusions from correctly calculated distributions [3] . Towards resolving this dispute, we present experimental results on the structure of mass-selected 4 He 3 and 3 He 4 He 2 trimers. Our experimental technique is based on femtosecond laser pulse ionization of the helium atoms constituting the trimer and subsequent imaging of the momentum vectors of the Coulomb exploding fragment ions using cold target recoil ion momentum spectoscropy (COLTRIMS) [23] , [24] (see Methods). Our experimental approach gives direct experimental access to the He–He distances and thus to the size of the trimer as well as to the bond angles. Size of the trimers The distribution of internuclear distances R between two 4 He atoms belonging to 4 He 3 is shown in Fig. 1 . The distribution extends from 3.3 to 12 Å (full width at half maximum). 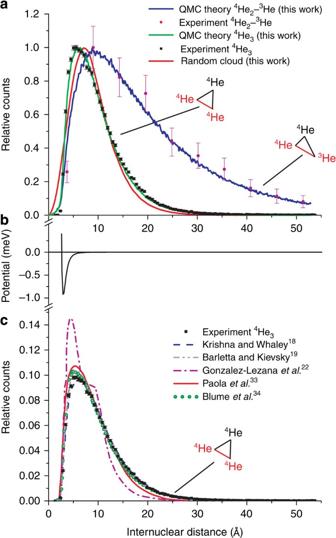Figure 1: Internuclear two-body distances. (a) Experimental distribution of the4He–4He distance of4He3and the4He–3He distances of3He4He2compared with QMC theory (this work) and a random cloud model (this work). Error bars result from the statistical errors. (b) He–He potential energy curve provided from the authors of ref.4. (c)4He–4He comparison with theoretical predictions. Figure 1 reveals a manifold of information: first, contrary to covalently bound molecules 4 He 3 clusters are (as van der Waals systems) basically empty, that is, the distance between the atoms is more than one order of magnitude larger than their diameter (which is only around 1 Å). Second, and even more important—and in this respect small He clusters differ from all other ground-state van der Waals systems—the size of the He trimer is not well defined. The width of the distribution is bigger than its mean value (which is 10.4 Å for 4 He 3 and 20.5 Å for 3 He 4 He 2 ) and it extends far beyond the minimum of the van der Waals interaction potential at 2.96 Å (see Fig. 1b ). Typically, the width of such a distribution stems from a superposition of vibrational ground and excited states. For the case of the helium trimer this is different. In 4 He 3 there is apart from the ground state only one other predicted vibrational state. That excited state, however, has not been observed so far [16] and is predicted to be an Efimov state with a size about 10 times larger than the ground state [9] , [25] . If it were present in our gas jet with the expansion parameters employed during the experiment, it would show up clearly in our data (see Methods). Therefore, the width of the distribution of internuclear distances results from the delocalized quantum nature of a single state. This quantum feature is uniquely strong for He 3 and becomes directly visible if one 4 He atom of the trimer is substituted by its isotope 3 He (see Fig. 1a ). Changing the mass does not effect the molecular potential. As an example, comparing the vibrational wave functions of H 2 and D 2 yields a slightly different mean value and a reduced width of the distribution of internuclear distances, just as expected from the altered vibrational kinematics. Figure 1 shows that the helium trimer isotope substitution leads to a much more dramatic change of the internuclear distances. The physical origin of this effect is twofold: the 25% reduction in mass leads to an increased zero-point energy and thus to a much lower binding energy. More important, however, is a second contribution: a significant part of the wave function extends beyond the classical turning point of the potential (which is at 9.5 Å for a binding energy of 1.2 μeV (ref. 11 )). This part of the vibrational wave function is therefore solely determined by tunnelling. Since the tunnelling probability depends exponentially upon the mass, the 3 He is able to tunnel into the barrier to much larger distances than 4 He. Figure 1: Internuclear two-body distances. ( a ) Experimental distribution of the 4 He– 4 He distance of 4 He 3 and the 4 He– 3 He distances of 3 He 4 He 2 compared with QMC theory (this work) and a random cloud model (this work). Error bars result from the statistical errors. ( b ) He–He potential energy curve provided from the authors of ref. 4 . ( c ) 4 He– 4 He comparison with theoretical predictions. Full size image In Fig. 1a , we compare the experimental distributions of internuclear distances to quantum Monte Carlo (QMC) simulations [26] using the TTY helium–helium potential [27] , which show excellent agreement (see Methods). Figure 1c compares our data to other published theoretical prediction. Within the experimental error bars all predictions perform extremely well with one exception, namely, the distribution obtained by González-Lezana et al. [22] Geometrical structure So far we have proven experimentally the highly diffuse shape of the trimer by investigating the internuclear distance between two atoms of the trimer. To yield a more direct access to the disputed geometry of the trimer, we considered only those events that stem from triple ionization and where we detected the vector momenta of the all three ions after Coulomb explosion. We have retrieved the initial spacial geometry from the measured momenta by employing Newton’s equations of motion. The obtained distribution of corner angles is shown in Fig. 2 . For a stiff van der Waals molecule such as Ne 3 (ref. 1 ), this distribution shows a narrow peak at 60°. A purely linear molecule would show peaks at 0 and 180°. For He 3, we find the distribution of angles to be extremely broad. 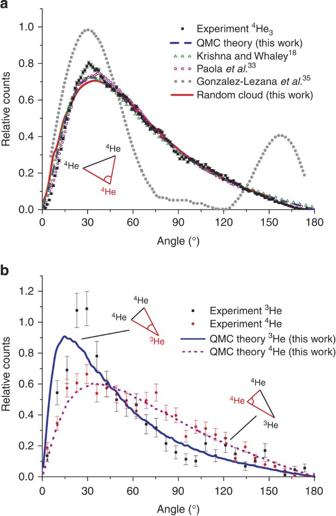Figure 2: Distribution of corner angles. (a) Distribution of the corner angle of4He3. The distribution of González-Lezana was obtained by transforming the cos(Θ) plot displayed in ref.35, weighting the probabiltiy with sin(Θ). (b) Corner angles of3He4He2at the4He atoms and at the3He atom. Error bars result from the statistical errors. Figure 2: Distribution of corner angles. ( a ) Distribution of the corner angle of 4 He 3 . The distribution of González-Lezana was obtained by transforming the cos(Θ) plot displayed in ref. 35 , weighting the probabiltiy with sin(Θ). ( b ) Corner angles of 3 He 4 He 2 at the 4 He atoms and at the 3 He atom. Error bars result from the statistical errors. Full size image Nevertheless, what does the distribution of one corner angle, shown in Fig. 2 , tell about the real shape of the trimer disputed in the literature? To answer this question, it is important to realize that any such distribution function is shaped by two factors: first, the phase space volume contributing to a particular interval of values and second, the few-body physics one aims to understand. To disentangle these two effects, it is helpful to compare the measurement with a distribution obtained from a simple model system for which we have a firm intuitive understanding. For this purpose, we use a completely structureless cloud made of randomly distributed points (see Methods). This cloud is homogeneously filled inside a sphere with a diameter of 4.3 Å and fades out exponentially from there (see Fig. 3a ). We randomly pick three points from this cloud and investigate the resulting triangles. The distribution of angles produced from such a homogenous random cloud almost perfectly coincides with that of the controversially discussed He 3 . 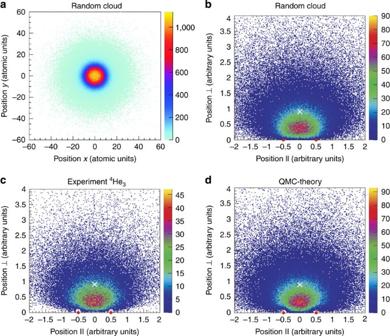Figure 3: Density distributions. (a) Density distribution of He atoms in a random cloud projected into thex– yplane. (b–d) Density distributions of the third particle in the case where the first two are fixed at the positions of the red dots. The random cloud model (b) yields, with an exception of the areas very close to the first and second particle, a distribnution that is very similar to the experimetal one (c) and to the one of the QMC calculations (d). The grey cross marks the position of the third particle for the case of a hypothetical equilateral triangle. Figure 3: Density distributions. ( a ) Density distribution of He atoms in a random cloud projected into the x– y plane. ( b – d ) Density distributions of the third particle in the case where the first two are fixed at the positions of the red dots. The random cloud model ( b ) yields, with an exception of the areas very close to the first and second particle, a distribnution that is very similar to the experimetal one ( c ) and to the one of the QMC calculations ( d ). The grey cross marks the position of the third particle for the case of a hypothetical equilateral triangle. Full size image To get an even better insight into the structure of the trimer, it is helpful to look at it in a two-dimensional histogram, as it provides a more intuitive picture of the shape. We chose a representation in which the trimer is rotated into a plane. The first and second particle, which are randomly chosen, are located on the negative and positive x axes and their distance is normalized to 1 (red dots in Fig. 3b–d ). The position of the third particle, normalized with the same normalization factor, is plotted on the positive y plane. As can be seen in Fig. 3 , the densitiy distribution of the third particle is highly diffuse. It does not show a maximum at the equilateral configuration (grey crosses) and also stretches far into the region of scalene geometry. Almost linear configurations are also present in the data, as isoscele geometries are. This lack of a rigid structure shows the unique charater of 4 He 3 and supports the conclusions already drawn from Figs 1 and 2 . The measured two-dimensional density distribution ( Fig. 3c ) is well reproduced by our elaborat quantum calculation but also by the simple random cloud model. Our results suggest that 4 He 3 is structureless, as our findings show that it adopts roughly as many structures of equilateral and linear triangular shape as a random cloud of appropriate size, demonstrating that the notion of equilibrium structure for this molecular system is ill defined [3] . This is, however, only true for the mono-isotopic 4 He 3 . In fact, the shape of the isotope-mixed 3 He 4 He 2 ( Fig. 2b ) is very different. The angle at the 3 He corner is much smaller than the angle in the 4 He corners of this triangle. The two 4 He atoms are closer together and the lighter 3 He is mainly found in the tunnelling region beyond the classical turning point. The mixed trimer thus forms an acute triangle. The He trimers studied here are few-body systems at the brink of universality. In the universality limit, the wave function of a few-body system does not depend anymore on the details of the potential and becomes scale invariant. As this limit is approached, a larger and larger part of the wave function is situated in the classically forbidden spatial region, which a particle can only access by quantum mechanical tunnelling. While for 4 He 3 the fraction of the wave function in this region is only small, the light isotope in 3 He 4 He 2 has already the biggest part of its probability density in the tunnelling region. Thus, we propose that 3 He 4 He 2 becomes a quantum halo state, similar to states that are well known in nuclear physics [14] , [28] , [29] . Because of the scale invariance, such few-body systems are important in nature across all the differently energy scales from nuclear physics to the physics of cold atoms. The imaging technology applied here opens a completely new observation window into this world of universal few-body systems. 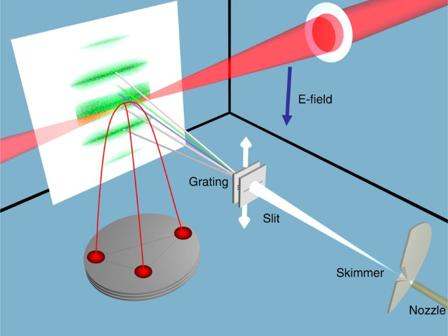Figure 4: Experimental set-up. Helium is expanded at 12 K at a driving pressure of 3 bar through a 5-μm nozzle to produce clusters. These are seperated by a 100 nm transmission diffraction grating. Behind the grating the first-order diffraction of the trimers is displayed in blue, the dimers in green. First-order monomers and the zero-order diffracted jet are shown in grey and illustrated on the screen in green. Dimers and trimers are not displayed on the screen because of their low intensity. Mass-selected clusters get ionized in a ~20 × 20 × 200 μm3laser focus. Fragments are guided on a position and time-sensitive detector by a homogeneous electric field. Experiment Figure 4 gives an overview of the present experiment. We combine mass selection by matter wave diffraction as pioneered by Toennies and Schöllkopf [15] with laser Coulomb explosion imaging using cold target recoil ion momentum spectoscropy (COLTRIMS) [23] , [24] . Figure 4: Experimental set-up. Helium is expanded at 12 K at a driving pressure of 3 bar through a 5-μm nozzle to produce clusters. These are seperated by a 100 nm transmission diffraction grating. Behind the grating the first-order diffraction of the trimers is displayed in blue, the dimers in green. First-order monomers and the zero-order diffracted jet are shown in grey and illustrated on the screen in green. Dimers and trimers are not displayed on the screen because of their low intensity. Mass-selected clusters get ionized in a ~20 × 20 × 200 μm 3 laser focus. Fragments are guided on a position and time-sensitive detector by a homogeneous electric field. Full size image The clusters are produced in a free-jet gas expansion [30] , [31] of pure 4 He (respectively, a mixture of 99% 3 He, 1% 4 He) source gas. A nozzle of 5 μm diameter was cooled down to 12 K at a driving pressure of 3 bar. This resulted in around 3–5% trimers (respectively, 0.1% isotopic trimers). About 49 cm downstream of the nozzle the beam was collimated by a slit of 25 μm right before a nanostructured diffraction grating of 100 nm grating period with an equal slit and bar width. As particles of all masses travel at the same velocity in the supersonic beam, different cluster masses lead to different deBroglie wavelengths and hence, become separated in angle behind the diffraction grating. Approximately 50 cm downstream of the grating, at the laser focus, the first-order diffraction peak of the trimers is separated by 600 μm from the zero-order beam, well separated from the first-order dimer peak at 900 μm, both having a FWHM of about 200 μm. Femtosecond laser pulses (~2 × 10 15 W cm −2 at 8 kHz, 40-fs pulse width (KMLabs Dragon)) are focused onto the beam of trimers. At this intensity, He single ionization is saturated and in the centre of the focus all three atoms of the trimer become singly ionized. In the outer region of the focal volume, however, the ionization probability per atom is not unity, and thus we obtain also events in which two out of the three atoms are ionized. The Coulomb exploding fragments are guided by a homogeneous electric field (15.25 V cm −1 ) onto a position- and time-sensitive micro channel plate detector with delay-line readout [32] . With the knowledge of time-of-flight, position on the detector, geometry of the setup and electric field the three-dimensional momentum vectors of all charged particles are obtained in coincidence. The trimer beam is very dilute resulting in a three ion coincidence rate of about 8 Hz. In contrast, the residual gas ionization rate was about 2 kHz at a vacuum pressure condition of 1.2 × 10 −11 mbar. For each event, we calculate the sum momentum of all ions. Since the photon momentum is neglegible on this scale, by momentum conservation the sum momentum of the ions for three charged particles is equal to the sum momentum of the electrons. It is typically<5 atomic units and hence much lower than the momenta from the Coulomb explosion. We use a gate on small ion sum momenta for background suppression. If only two ions are produced, the remaining neutral atom does not participate in the Coulomb explosion and has only negligible momentum, while the two ions are emitted back-to-back. This allows us to clearly separate a two-ion-one-neutral event from those events where three atoms were ionized and Coulomb exploded with large momenta, but only two were detected. From these two-body Coulomb explosion events we obtain the data shown in Fig. 1 . The internuclear distance R between the two ions corresponds to a potential energy of 1/ R . As the ions fly apart, driven by the mutual Coulomb repulsion, their potential energy is converted to kinetic energy release of the ion pair (KER 2 ), which is measured. Thus, the internuclear distance at the instant of ionization is given by R =1/KER 2 (atomic units are used throughout this paper unless stated otherwise). For those events where all three atoms were ionized by the laser pulse, the momentum of the three ions is given by their mutual Coulomb repulsion. The potential energy at the instant of ionization is converted into a measurable fragment kinetic energy release for a three-body Coulomb explosion ( KER 3 ) given by where R ij is the distance between ions i and j . The measured KER 3 distributions are shown in Fig. 5 . Compared with other van der Waals clusters the distributions of Helium are very broad. This finding for three-body Coulomb explosion is in line with the finding from two-body fragmentation shown in Fig. 1 . 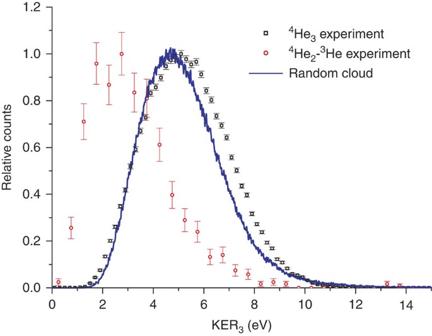Figure 5: Kinetic energy releases. Sum of the kinetic energies of the He ions from ionization of each of the atoms of mass-selected4He3and3He4He2by a femtosecond laser pulse. Error bars result from the statistical errors. Figure 5: Kinetic energy releases. Sum of the kinetic energies of the He ions from ionization of each of the atoms of mass-selected 4 He 3 and 3 He 4 He 2 by a femtosecond laser pulse. Error bars result from the statistical errors. Full size image We emphasize that in Fig. 5 the presence of the predicted Efimov state of 4 He 3 would appear as an additional peak between 0 and 1.5 eV as this state is predicted to be about 10 times more extended than the 4 He 3 vibrational ground state [16] . From the measured three momentum vectors of these triple ionization events, the distribution of angles shown in Fig. 2 are generated by solving Newton’s equation of motion. QMC theory In the QMC calculation, we described the ground-state wave functions of the helium trimers with a pair-product form where R ij is the distance between the two atoms and φ ij ( R ij ) is the pair function describing their interaction. In the case of the 4 He 3 system all the pair functions must be equal for symmetry reasons, while for the 3 He 4 He 2 trimer only the pair functions for the 3 He– 4 He interactions must be equal while the 4 He– 4 He pair function can be independently optimized. We employed the widely used pair function. The variational parameters have been optimized using the variational Monte Carlo method [26] . The optimized wave functions have been subsequently employed in diffusion Monte Carlo [26] simulations to sample the exact ground-state wave functions, from which it is possible to estimate the desired geometrical properties. Random cloud model In the random cloud model shown in Fig. 3a , we created a three-dimensional random cloud of individual particles with a constant probability density up to a radius of R =4.3 Å. Outside this radius the probability density decreases as exp(− κ · r ), with κ =0.16. This three-dimensional single-particle probability density serves as an input for a random generator, with which we pick a large number of individual geometries of trimers. For each individual trimer geometry we randomly pick three times a particle coordinate with the individual probability given by the random cloud just described. The three picks for each individual trimer are completely independent, there is no correlation between the three particles. R and κ are chosen such that the results fit to the data presented in Fig. 2 . The random cloud model does not include any short-range correlations. Therefore, it contains also unphysical small distances between the two particles. This can, for example, be seen in Fig. 3 . The experimental data and the QMC calculation show no density of particle three in the regions close to one of the two other particles, because of the repulsive nature of the He–He interaction potential at small distances. This feature is absent in the random cloud model. The good agreement that this simple model yields with the full calculation as well as the measured data shows that the weight of these small interatomic distances to the total distribution is very small. The repulsive inner region of the two-body potential does determine the overall size of the system, which in the random cloud model is determined by the two free parameters R and κ . How to cite this article : Voigtsberger, J. et al. Imaging the structure of the trimer systems 4 He 3 and 3 He 4 He 2 . Nat. Commun. 5:5765 doi: 10.1038/ncomms6765 (2014).